Correlated electron–hole plasma in organometal perovskites Organic–inorganic perovskites are a class of solution-processed semiconductors holding promise for the realization of low-cost efficient solar cells and on-chip lasers. Despite the recent attention they have attracted, fundamental aspects of the photophysics underlying device operation still remain elusive. Here we use photoluminescence and transmission spectroscopy to show that photoexcitations give rise to a conducting plasma of unbound but Coulomb-correlated electron–hole pairs at all excitations of interest for light-energy conversion and stimulated optical amplification. The conductive nature of the photoexcited plasma has crucial consequences for perovskite-based devices: in solar cells, it ensures efficient charge separation and ambipolar transport while, concerning lasing, it provides a low threshold for light amplification and justifies a favourable outlook for the demonstration of an electrically driven laser. We find a significant trap density, whose cross-section for carrier capture is however low, yielding a minor impact on device performance. Organic–inorganic perovskite semiconductors combine the advantages of low-cost solution processability together with efficient charge transport, strong light absorption, favourable emission properties and optical gap tunability across the entire visible spectrum [1] , [2] , [3] , [4] , [5] , [6] , [7] , [8] , [9] , [10] , [11] , [12] , [13] , [14] , [15] , [16] . As a matter of fact, there exist only a few examples of materials in nature showing both good carrier transport properties and controllable optical characteristics, and most of them do not match the demand of low-cost processing. Photovoltaic devices based on thin films of organometal perovskites deposited by simple spin-coating techniques outperform other solution-processed solar cells. At the same time, perovskites can be also used as gain medium for lasing, featuring low threshold densities for on-chip light sources [17] , [18] . Understanding the excited-state properties of this class of materials is an important issue [19] , [20] , [21] , [22] , [23] , [24] , [25] , [26] , [27] , [28] . Long-range Coulomb interaction between optically or electrically injected charges has a simple form, but depending on the materials and the excitation regimes, it can give rise to a large variety of exotic excited states in organic and inorganic semiconductors. The interaction strength, which can be affected by screening and quantum-mechanical effects, is often measured by the binding energy of excitons, the bound state of an electron–hole pair. Light emission from perovskite films occurs close to the first excitonic peak observed in absorption, and so does stimulated emission [17] , [18] . It therefore appears natural that most of the reports published so far discuss the basic photophysical properties in terms of excitons and their dynamics. Exciton binding energies, E b , in the range of 20–60 meV have been reported [21] , [29] , [30] , [31] . An exciton is a charge-neutral state that needs to be split into free opposite charges, for example, in a type II heterojunction, to yield a current flow. Whether the excited state of perovskite crystals is made by an insulating exciton gas, as typically occurs in organic semiconductors, or by a conducting plasma of ionized exciton particles, as usually happens in low-gap inorganic semiconductors at room temperature, is essential to design photovoltaic devices with improved performances. The microscopic processes involved in the stimulated light emission in a semiconductor are also different if an exciton gas or a plasma of unbound electrons and holes are involved, primarily due to the different way to accumulate for population inversion in Bose and Fermi distributions. In organics, an incoherent exciton population is generated following optical excitation; stimulated emission requires the annihilation of an exciton and the generation of a ground state vibration, very similar to a molecular three-level system [32] , [33] . In inorganic semiconductors, light amplification at room temperature mostly occurs from electron–hole recombination in a conducting plasma. The excitation threshold for lasing requires the accumulation of electrons and holes, respectively, at the bottom and top of the conduction and valence bands to establish a population inversion, likewise to an atomic two-level system [34] , [35] . The perovskite being a hybrid, partly organic and partly inorganic compound, it is not clear in principle whether the excited-state dynamics will be dominated by excitonic effects, as in organic semiconductors, or by an electron–hole plasma, as happens in the inorganic compounds. Here we investigate the nature of the excited state in organometal halide perovskites for different excitation conditions, ranging from carrier densities lower than what is produced under solar illumination to higher than what is required to sustain optical amplification. The exciton binding energy is accurately determined by analyzing the excitonic enhancement of the absorption edge in the framework of the Elliot’s theory of Wannier excitons [36] , resulting in E b =25±3 meV, a value comparable to the thermal energy at room temperature. Excitonic correlation is found to enhance optical absorption at the band edge and also affect optical emission, as the photoluminescence (PL) spectrum consists of a slightly asymmetric line peaked close to the exciton resonance. Such properties at room temperature are typical of an organic semiconductor. However, the analysis of the transient PL as a function of the injected charge density tells a different story: the rate of spontaneous photon emission scales quadratically with n 0 up to the electron–hole densities required to observe optical gain ( n las ~2 × 10 18 cm −3 ; ref. 17 ). These experimental results indicate that the injected electron–hole gas thermalizes at the conduction and valence band extremes to form an ionized electron–hole plasma and a negligible exciton population, even for excitation regimes for which thermodynamic considerations would predict a transition to an insulating excitonic gas. Such photophysics resembles the excited-state properties of model inorganic semiconductors with direct bandgap energy and small exciton binding energies. We were also able to investigate the influence of trap states, which are expected to be plentiful in a solution-processed, self-assembled crystal. We provide evidence that, even if their density is not negligible, traps have a low capture cross-section and play a minor role both for photovoltaic energy conversion and light amplification. Band-edge excitations in trihalide perovskite films We prepared films of two different perovskite materials, namely pure methylammonium lead iodide CH 3 NH 3 PbI 3 (MAPbI 3 ) and mixed CH 3 NH 3 PbI 3− x Cl x (MAPbI 3− x Cl x ), using the procedures described in the Methods section. The film X-ray diffraction patterns are as shown in Supplementary Fig. 1 . 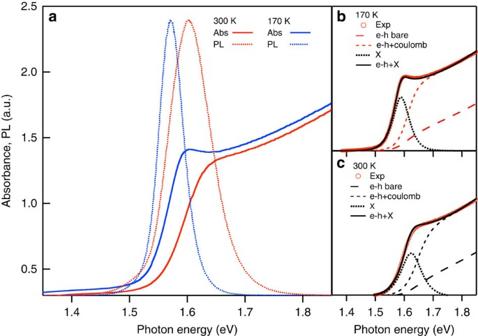Figure 1: Absorption and photoluminescence spectra in trihalide perovskite films. (a) Visible–near-infrared absorption (continuous line) and luminescence (dashed line) spectra of a MAPbI3film (thickness, 800 nm) recorded at 300 and 170 K. Spontaneous emission was excited by a green laser (λ=532 nm) operating in continuous wave (cw). (b,c) Continuous lines: theoretical fits to the experimental absorption spectra at 170 and 300 K, respectively. Excitonic and band-to-band oscillator strengths are calculated taking into account Coulomb interaction according to Elliott’s theory of Wannier excitons. Dotted lines: exciton transitions. Short-dashed (long-dashed) lines: band-to-band contributions with (without) the inclusion of Coulomb interactions. Exciton binding energy: 25±3 meV.Eg=1.612 eV, Γ=0.023 eV and 1.647 eV, Γ=0.031 eV at 170 and 300 K, respectively. Figure 1 shows the absorbance spectrum of a MAPbI 3 film near the optical gap at 170 and 300 K. Similar results were obtained in MAPbI 3− x Cl x mixed halide perovskite films (see Supplementary Fig. 2 ). At low temperature, the lowest excitonic transition manifests itself as a weak peak at the absorption edge. Owing to the significant thermal-induced line broadening, the bound-exciton and band-to-band transitions are spectrally unresolved. Measurements were not extended below ~160 K, as the crystal undergoes a phase transition from the tetragonal to the orthorhombic phase that prevents the observation of narrower spectral lines in the tetragonal structure [37] . Figure 1: Absorption and photoluminescence spectra in trihalide perovskite films. ( a ) Visible–near-infrared absorption (continuous line) and luminescence (dashed line) spectra of a MAPbI 3 film (thickness, 800 nm) recorded at 300 and 170 K. Spontaneous emission was excited by a green laser ( λ =532 nm) operating in continuous wave (cw). ( b , c ) Continuous lines: theoretical fits to the experimental absorption spectra at 170 and 300 K, respectively. Excitonic and band-to-band oscillator strengths are calculated taking into account Coulomb interaction according to Elliott’s theory of Wannier excitons. Dotted lines: exciton transitions. Short-dashed (long-dashed) lines: band-to-band contributions with (without) the inclusion of Coulomb interactions. Exciton binding energy: 25±3 meV. E g =1.612 eV, Γ=0.023 eV and 1.647 eV, Γ=0.031 eV at 170 and 300 K, respectively. Full size image The PL spectrum consists of a single line slightly shifted to the red with respect to the excitonic absorption peak. As shown in Supplementary Fig. 3 , the energy shift is mostly caused by self-absorption due to the finite thickness of the film. The shape of the emission corrected for self-absorption and the emission in thinner films is almost coincident with the excitonic resonance, while the shape is slightly asymmetric towards the higher energy side. These results point to the intrinsic nature of the emitting species. The emission narrows and blueshifts with decreasing temperature, following the shift in the absorption spectrum. Numerical modelling of band-edge absorption We modelled the absorption coefficient α ( ħω ) near the band edge in the framework of the Elliot’s theory of Wannier excitons [36] : This equation is valid for bulk semiconductors with exciton binding energies much smaller than the bandgap (Wannier excitons) and was successfully applied in literature to describe optical transitions to bound and ionized excitonic states in model inorganic semiconductors, such as GaAs and GaP [38] , [39] . μ cv is the transition dipole moment; ℏ ω the photon energy. α ( ħω ) is proportional to the weighted density of electron–hole pair states, with the weight provided by the probability for an electron and a hole to be at the same position | ϕ j ( r =0)| 2 , where ϕ j represents the exciton wavefunction of bound and unbound states. The first term in the last expression of equation 1 describes transitions to bound states with energy , while the second term refers to continuum states with energies above the bandgap E g ; δ ( x ) and θ ( x ) are the Dirac-delta and the Heaviside step functions, respectively. The absorption in the continuum spectrum does not simply follow the square root dependence of the density of states on energy , as expected for bare band-to-band transitions between uncorrelated electron and hole particles. The excitonic enhancement of the optical density of states depends on the strength of the Coulomb interaction, through the exciton binding energy, and provides a measure of the degree of electron–hole correlation. We convoluted α ( ℏ ω ) with a secant hyperbolic function of width Γ to simulate line broadening and introduced a non-parabolic band dispersion. We fitted the absorption spectrum at 300 and 170 K, using E B and Γ as free parameters. Details of the analysis are presented in Supplementary Methods . Because of strong light diffusion in mixed halide perovskites, the fit analysis was limited to the MAPbI 3 film. A satisfactory agreement with experiments at both temperatures was found for E B =25±3 meV (see Supplementary Fig. 4 to visualize how the absorption lineshape depends on E B ). The small binding energy, comparable to the thermal energy (26 meV), is likely due the large dielectric constant of these materials [29] , [30] and is intermediate between the large binding energy of Frenkel excitons in organic semiconductors (typically >100 meV; ref. 40 ) and the low value of Wannier excitons in inorganic semiconductor with near-infrared bandgaps (typically <10 meV; ref. 34 ). The comparison between experiment and theory shows the crucial role of electron–hole correlation effects in optical transitions near the band edge, even at room temperature. The absorption coefficient of correlated electron–hole pairs is over a factor of two larger than that one calculated for uncorrelated free carriers in a wide spectral window above the bandgap. Transient PL spectroscopy We then turned to ultrafast optical spectroscopy, particularly to time-resolved PL, to investigate the effect of excitonic correlations on the excited-state relaxation dynamics. 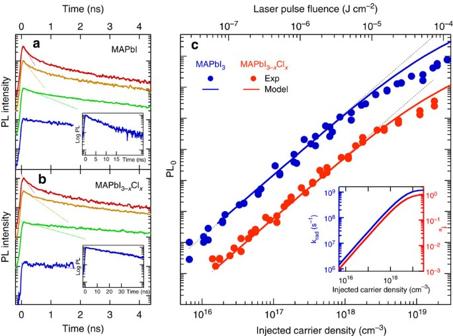Figure 2: Transient photoluminescence spectroscopy in trihalide perovskites: bound versus unbound electron–hole pair states. (a,b) Transient photoluminescence signal as a function of the injected electron–hole pair density at the film surface (n0). Straight lines in the semi-logarithmic plot represent an exponential fit to the initial decay of the photoluminescence signal. Photoluminescence was excited by 150-fs-long laser pulses with a repetition rate of 1 kHz and 3.18 eV photon energy. At this light wavelength, the trihalide perovskite absorption coefficient is 1.2 × 105cm−1. (a) From top to bottom:n0=1.2 × 1019cm−3, 3.9 × 1018cm−3, 1.2 × 1018cm−3and 1.9 × 1017cm−3. (b) From top to bottom:n0=1.1 × 1019cm−3, 3.5 × 1018cm−3, 1.1 × 1018cm−3, 1.7 × 1017cm−3. (c) Photoluminescence emission intensity estimated att=0 (PL0) as a function of injected electron–hole density (lower axis) and laser pulse fluence (upper axis). For laser pulse fluences >10−4μJ cm−2the PL0value could not be extracted from measured decays, as they were much faster than the experimental resolution. The quadratic dependence is shown by the black-dotted lines as a guide for eyes. Continuous lines: PL0intensities calculated according to the Kubo–Martin–Schwinger relation (equation (2)) for the radiative recombination of ionized plasma in a semiconductor. Simulations consider the exponential spatial profile of the electron–hole density created by laser pulses. PL0is calculated by summing the spontaneous emission intensity emitted by plasma along the light absorption path. Deviation from the quadratic law stems from band filling and many-body effects. Inset: calculated spontaneous photon emission per electron–hole pair (krad, blue line) and occupation number of the lowest electron (hole) states in a non-interacting plasma based on Fermi–Dirac statistics (fe(h), red line). Figure 2 reports the PL decays of perovskite films excited by sub-picosecond laser pulses and detected by a streak camera (see Methods for details); Figure 2a,b shows the PL decay traces measured with the streak camera for the two perovskite films, MAPbI 3 and MAPbI 3− x Cl x , respectively. Following excitation, carriers quickly thermalize to the extremes of the conduction and valence bands. The optically injected electron–hole pair density n 0 at the film surface was estimated by multiplying the laser pulse photon fluence times the film absorption coefficient and ranged from ~10 16 to ~10 19 cm −3 . In this carrier density range, the transient emission spectrum is always peaked at the exciton resonance, ℏ ω = E X (spectra shown in Supplementary Fig. 5 ). However, the exciton binding energy is small, and the high-energy side of the PL spectrum overlaps with the expected energies of band-to-band transitions. Under all excitation conditions and for all samples, the PL signal rises instantaneously; if an exciton population is formed, this process takes place within the temporal resolution of our experimental set-up, ~60 ps. 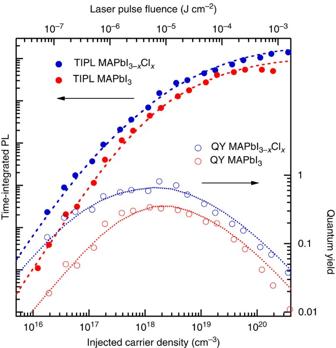Figure 3: Photoluminescence quantum yield. Time-integrated photoluminescence signals (TIPL) for the two perovskite samples (MAPbI3red dots, MAPbI3−xClxblue dots) are plotted on the left axis as a function of the injected carrier density. As a reference, the laser pulse fluence directly measured in the experiments is also reported on the top axis. The dashed lines correspond to the prediction from a rate equation model accounting for the main relaxation channels for electrons and holes. Simulations take into account the exponential spatial profile of the electron–hole density created by laser pulses. The initial dependence on the injected carrier density is superlinear, up to 1018cm−3, then the slopes become sublinear. The injected carrier density is calculated multiplying the laser pulse photon fluence by the absorption coefficient of the films. The emission quantum yields (QY) are calculated as TIPL/Φ, whereΦis the laser pulse fluence, and also shown against the right axis. Initially the QY grows with fluence for both films, as the bimolecular recombination becomes faster and a growing fraction of the injected excitations recombine radiatively, instead of being trapped. At excitations >1019cm−3, non-radiative Auger processes dominate. The absolute QY is scaled to match theoretical predictions. The maximum QY values are ~30% for MAPbI3and >70% for MAPbI3−xClx. The dotted lines represent predictions from the same-rate equation model employed for the TIPL. The very good agreement between model and data indicates that the main photophysical processes are accounted for in the model. Figure 3c reports the PL signal, PL 0 just after laser excitation and before electronic states are depopulated by slow recombination processes. The quantity PL 0 is therefore proportional to the rate of spontaneous photon emission per unit of volume, R ( n ). Up to pulse fluences Φ ~10 μJ cm −2 , PL 0 scales quadratically in the laser pulse fluence and therefore in the injected carrier density n 0 . Such scaling is expected from the bimolecular emission by a gas of unbound electron–hole pairs [41] , where the radiative recombination rate is proportional to the probability of an electron meeting a hole and therefore to the product of electron and hole densities: . Remarkably, our experimental evidence indicates that exciton correlation greatly enhances light absorption in organometal halide perovskites, but the resulting optical excitations are unbound and move freely in the crystal. In other words, bound-exciton states exist, but they are not populated. PL 0 tends to saturate for pulse fluences higher than Φ~ 10 μJ cm −2 , corresponding to an injected saturation density n sat ~2.5 × 10 18 cm −3 , a value comparable to the threshold density for lasing, n las , reported in literature [17] . Figure 2: Transient photoluminescence spectroscopy in trihalide perovskites: bound versus unbound electron–hole pair states. ( a , b ) Transient photoluminescence signal as a function of the injected electron–hole pair density at the film surface ( n 0 ). Straight lines in the semi-logarithmic plot represent an exponential fit to the initial decay of the photoluminescence signal. Photoluminescence was excited by 150-fs-long laser pulses with a repetition rate of 1 kHz and 3.18 eV photon energy. At this light wavelength, the trihalide perovskite absorption coefficient is 1.2 × 10 5 cm −1 . ( a ) From top to bottom: n 0 =1.2 × 10 19 cm −3 , 3.9 × 10 18 cm −3 , 1.2 × 10 18 cm −3 and 1.9 × 10 17 cm −3 . ( b ) From top to bottom: n 0 =1.1 × 10 19 cm −3 , 3.5 × 10 18 cm −3 , 1.1 × 10 18 cm −3 , 1.7 × 10 17 cm −3 . ( c ) Photoluminescence emission intensity estimated at t =0 (PL 0 ) as a function of injected electron–hole density (lower axis) and laser pulse fluence (upper axis). For laser pulse fluences >10 −4 μJ cm −2 the PL 0 value could not be extracted from measured decays, as they were much faster than the experimental resolution. The quadratic dependence is shown by the black-dotted lines as a guide for eyes. Continuous lines: PL 0 intensities calculated according to the Kubo–Martin–Schwinger relation (equation (2)) for the radiative recombination of ionized plasma in a semiconductor. Simulations consider the exponential spatial profile of the electron–hole density created by laser pulses. PL 0 is calculated by summing the spontaneous emission intensity emitted by plasma along the light absorption path. Deviation from the quadratic law stems from band filling and many-body effects. Inset: calculated spontaneous photon emission per electron–hole pair ( k rad , blue line) and occupation number of the lowest electron (hole) states in a non-interacting plasma based on Fermi–Dirac statistics ( f e(h) , red line). Full size image Figure 3: Photoluminescence quantum yield. Time-integrated photoluminescence signals (TIPL) for the two perovskite samples (MAPbI 3 red dots, MAPbI 3− x Cl x blue dots) are plotted on the left axis as a function of the injected carrier density. As a reference, the laser pulse fluence directly measured in the experiments is also reported on the top axis. The dashed lines correspond to the prediction from a rate equation model accounting for the main relaxation channels for electrons and holes. Simulations take into account the exponential spatial profile of the electron–hole density created by laser pulses. The initial dependence on the injected carrier density is superlinear, up to 10 18 cm −3 , then the slopes become sublinear. The injected carrier density is calculated multiplying the laser pulse photon fluence by the absorption coefficient of the films. The emission quantum yields (QY) are calculated as TIPL/ Φ , where Φ is the laser pulse fluence, and also shown against the right axis. Initially the QY grows with fluence for both films, as the bimolecular recombination becomes faster and a growing fraction of the injected excitations recombine radiatively, instead of being trapped. At excitations >10 19 cm −3 , non-radiative Auger processes dominate. The absolute QY is scaled to match theoretical predictions. The maximum QY values are ~30% for MAPbI 3 and >70% for MAPbI 3− x Cl x . The dotted lines represent predictions from the same-rate equation model employed for the TIPL. The very good agreement between model and data indicates that the main photophysical processes are accounted for in the model. Full size image In the following, we investigate the electron–hole recombination by studying the dependence on the pulse fluence of (i) the temporal-integrated PL intensity (TIPL); (ii) the PL quantum yield QY and (iii) the initial PL decay rate . Figure 3 shows the TIPL intensity and the relative QY for the same films investigated in Fig. 2 . The TIPL grows quadratically until n 0 ~10 17 cm −3 , before showing some saturation at higher fluences. Correspondingly the QY, calculated as TIPL/ Φ , grows linearly, then saturates, and for n 0 > n sat , it decreases. This nonlinear behaviour can be ascribed to the interplay between density-dependent radiative and non-radiative recombination mechanisms. We rationalize the recombination kinetics as follows: for n 0 <10 17 cm −3 , carrier trapping is faster than radiative recombination; the increase of the QY with pulse fluence is then associated with the increase of the bimolecular radiative recombination rate. When this latter becomes faster than trapping ( n 0 >10 17 cm −3 ), the QY saturates. If the injected electron–hole population is further increased, n 0 > n sat , density-dependent non-radiative processes become more and more important and eventually dominate, causing the decrease of the QY. PL decay rates are also sensitive to the recombination dynamics. In Fig. 4 are shown the initial decay rates of the PL signal, extracted from the decays in Fig. 2a,b . The PL signal becomes faster for increasing n 0 , indicating the activation of density-dependent recombination mechanisms. k PL is similar in both samples and shows a remarkable increase for injected population densities >10 17 cm −3 . For n 0 ~10 19 cm −3 , k PL ~10 10 s −1 . It should be noted that differs from the average PL lifetime τ obtained by fitting the PL decay with a single exponential. We found that τ =9 ns and 80 ns for MAPbI 3− x Cl x and MAPbI 3 , respectively. Although the average PL lifetimes of the films are different, the early-time nonlinear decays are quite similar, as shown in Fig. 4 . These findings indicate that the initial density-dependent decay of the PL signal is caused by intrinsic nonlinear processes, while the longer-time decay is dictated by extrinsic effects, such as traps and defects. 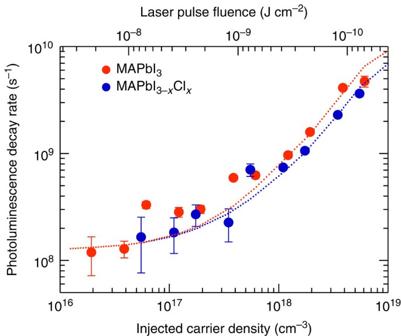Figure 4: Photoluminescence decay rates. The decay rates for the transient photoluminescence signal decays are plotted as a function of the injected carrier density (or laser pulse fluence on top axis). The rates, defined asare extracted from the data inFig. 2a,b. Such rates represent therefore the very initial decay and should not be mistaken for the average photoluminescence decay rate obtained by fitting the entire decay with an exponential function. The error bars represent the s.d. from a least square fit to an exponential decay and are reported only when they exceed the size of the marker. Remarkably, the rates are very similar for the two perovskites (although the average exponential decay rates are significantly different) and grow together for growing injected carrier densities. We infer that such rates measure the intrinsic density-dependent bimolecular and Auger recombination processes. The dotted lines represent the outcome of the rate equation model: also in this case the agreement with the experiment is satisfactory. Experimental and theoretical decay rates represent an exponential fit to the initial photoluminescence transients, carried out in the same time-window for experiments and simulations. The exponential spatial profile of the electron–hole density created by laser pulses is accounted for in the model simulations. Figure 4: Photoluminescence decay rates. The decay rates for the transient photoluminescence signal decays are plotted as a function of the injected carrier density (or laser pulse fluence on top axis). The rates, defined as are extracted from the data in Fig. 2a,b . Such rates represent therefore the very initial decay and should not be mistaken for the average photoluminescence decay rate obtained by fitting the entire decay with an exponential function. The error bars represent the s.d. from a least square fit to an exponential decay and are reported only when they exceed the size of the marker. Remarkably, the rates are very similar for the two perovskites (although the average exponential decay rates are significantly different) and grow together for growing injected carrier densities. We infer that such rates measure the intrinsic density-dependent bimolecular and Auger recombination processes. The dotted lines represent the outcome of the rate equation model: also in this case the agreement with the experiment is satisfactory. Experimental and theoretical decay rates represent an exponential fit to the initial photoluminescence transients, carried out in the same time-window for experiments and simulations. The exponential spatial profile of the electron–hole density created by laser pulses is accounted for in the model simulations. Full size image Numerical modelling of radiative recombination processes Driven by the experimental observations that the majority of the electron–hole pairs are unbound, we started estimating the radiative emission properties of a non-interacting electron–hole gas. In analogy with the Einstein’s relation connecting absorption and emission coefficients in atomic physics, the rate of spontaneous photon emission per unit volume, R ( n ), and the absorption coefficient in a semiconductor are connected via the so called Kubo–Martin–Schwinger relation [42] , [43] : where n r is the index of refraction, is the Bose function and μ the chemical potential of the photoexcited electron–hole plasma. The right hand side of equation 2) neglects many-body interactions and bound-exciton states, but it includes band filling effects through the product of the Fermi distributions of electrons and holes, f e ( ω ) f h ( ω ) (ref. 44 ). α 0 ( ω ) is thus the absorption coefficient of the continuum states for n =0. In Fig. 2c , we report three physical quantities of interest as a function of the plasma density: in the inset, the occupation probability of the lowest energy electron or hole states, f e(h) and the rate of spontaneous photon emission per electron–hole pair, namely ; in the main panel R , rescaled to match PL 0 at low pulse fluences. Let’s restrict the analysis for the sake of simplicity to the radiative recombination of one kind of carrier, electrons. In the dilute plasma regime, ( f e(h) ≪ 1), the rate of radiative electron recombination is proportional to the probability ( f h ∝ n ) to find a hole: k rad = k b n h = k b n . Therefore, k rad scales linearly with n , while the PL intensity grows as the square of the excitation density n : PL 0 ∝ R = k rad n = k b n 2 , where k b is the bimolecular decay constant, whose value was extracted from the experimental absorption data [19] : k b =2.6 × 10 −10 cm 3 s −1 . The scaling with the excitation density changes when occupation probability of the electron and hole states at the band edge is not anymore negligible, for n >10 18 cm −3 ( f e(h) >0.1). For n >10 19 cm −3 , f e(h) ~1 and the radiative recombination process becomes monomolecular, k rad = k sat =1.2·10 9 s −1 while PL 0 ∝ R = k sat n scales linearly. The model predicts the deviation from a quadratic behaviour of PL 0 at the electron–hole density observed experimentally, n ~ n sat . The predicted PL 0 saturation turns out to be slightly underestimated with respect to the experimental observation, which we interpret as a signature of many-body effects weakening the excitonic enhancement with respect to the low-excitation regime. Such many-body effects, however, do not significantly affect the transition energy of the exciton resonance, as observed in the transient spectra reported in Supplementary Fig. 5 . We speculate that the two expected effects of many-body interactions, namely redshift of the bandgap and reduction of the exciton binding energy, compensate for each other as observed in other semiconductors and predicted theoretically [44] . After analyzing the initial decay rates, we then proceeded to simulate the time integral of PL, namely TIPL and the QY as a function of the pulse fluence (reported in Fig. 3 ). We solved the rate (equations (2) and (3)) for the carrier population and the PL, in which we included (i) the radiative recombination rate taken from equation (2), (ii) the electron–hole annihilation rate via non-radiative Auger processes, proportional to γn 3 and (iii) a monomolecular decay k t n to describe carrier trapping. The monomolecular decay constant k t was tuned to reproduce the mean PL lifetime at low intensities. The only adjustable parameter to reproduce the experimental TIPL and QY was γ , which was set to 2 × 10 −28 cm 6 s −1 and 4 × 10 −28 cm 6 s −1 for MAPbI 3− x Cl x and MAPbI 3 , respectively [19] . The agreement with the experiment highlighted in Fig. 3 is satisfactory. The calculated QY reaches the remarkable values of 0.7 and 0.4 for the mixed and pure halide perovskites, respectively [18] . As the radiative recombination rate increases with carrier density, the QY is found to be very large for plasma densities at which optical gain can be achieved. This fact is promising for obtaining lasing action under optical, and possibly electrical, excitation in continuous wave (cw). The same nonlinear recombination parameters used for evaluating the integrated PL intensity and the emission quantum yield were also used to calculate the initial decay rate k PL in Fig. 4 , yielding again a good agreement with experiments. In this case, the monomolecular decay rate was fixed from the low-density decay rate of the PL in the 0–5 ns time range of interest. This is not in contrast with the trapping constant used to fit the QY and the TIPL signal. As charge trapping results from a carrier diffusive process, the trapping rate is not expected to be constant, but to slow down with time leading to a non-exponential PL decay [45] , [46] , [47] . Steady-state PL spectroscopy Transient PL is a valuable tool to sort the excited-state relaxation processes and determine their rates. Devices employing perovskite films are, however, expected to work under steady-state conditions, being the continuous operation of a solar cell or an optical emitter. Therefore, we verified our understanding of the photophysical processes against the steady-state PL intensity versus the continuous-wave excitation intensity, as reported in Fig. 5a . Laser intensity ranges over eight orders of magnitude, with the lowest intensity, I =10 −4 W cm −2 , one thousand times weaker than standard sunlight intensity, 0.1 W cm −2 , while the highest excitation values, I =10 4 W cm −2 , are of interest for the potential use of perovskite films as the active mediums for lasing. The PL intensity follows a 3/2 power law over more than five orders of magnitude in the excitation intensity. The power law indicates that under cw excitation, the electron–hole population is not governed by radiative bimolecular recombination alone. In this case, a linear dependence would be expected, as all recombination processes would be radiative. The observed PL response points to specific intra-gap states that act as traps for electrons or holes. 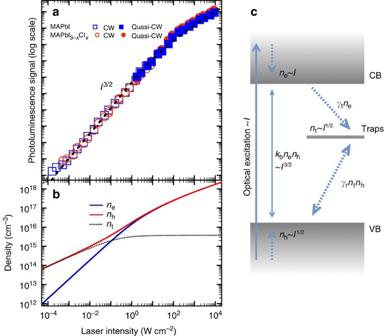Figure 5: Steady-state photoluminescence. (a) shows the photoluminescence signal as a function of the intensity of the exciting laser. The empty circles represent the measurements obtained with a cw Nd:Yag 532 nm laser; the filled circles are instead measured in quasi-cw conditions, exciting the samples with 300-ns-long laser pulses from a Q-switched 527 nm Nd:Ylf laser; the pulse duration is much longer than all the relevant relaxation rates, so that steady-state condition are expected to be achieved during laser excitation. The PL signal grows asI3/2for a wide range of excitations. Investigations were extended from laser intensities much lower than the solar one, to intensities large enough to create population inversion and optical gain. The unusual 3/2 power law is attributed to intra-gap trap states trapping either electrons or holes, but not both of them. Dashed-line shows the results of the trap model, under the assumption that electrons are the trapped species. Simulations consider the exponential spatial profile of the electron–hole density created by laser pulses as described in the legend ofFig. 2. Inb, the red line represents the hole densitynh, the blue one is the electron densityne, the dotted line is the density of filled trapsnt. As the excitation intensity grows the traps are filled, until the density of electrons and holes is large enough that the bimolecular recombination becomes faster than the trapping rate, therefore stopping the accumulation of electrons in the traps.cshows a sketch of the relaxation of optical excitations under steady-state conditions (VB and CB mark the valence and conduction bands, respectively). Figure 5: Steady-state photoluminescence. ( a ) shows the photoluminescence signal as a function of the intensity of the exciting laser. The empty circles represent the measurements obtained with a cw Nd:Yag 532 nm laser; the filled circles are instead measured in quasi-cw conditions, exciting the samples with 300-ns-long laser pulses from a Q-switched 527 nm Nd:Ylf laser; the pulse duration is much longer than all the relevant relaxation rates, so that steady-state condition are expected to be achieved during laser excitation. The PL signal grows as I 3/2 for a wide range of excitations. Investigations were extended from laser intensities much lower than the solar one, to intensities large enough to create population inversion and optical gain. The unusual 3/2 power law is attributed to intra-gap trap states trapping either electrons or holes, but not both of them. Dashed-line shows the results of the trap model, under the assumption that electrons are the trapped species. Simulations consider the exponential spatial profile of the electron–hole density created by laser pulses as described in the legend of Fig. 2 . In b , the red line represents the hole density n h , the blue one is the electron density n e , the dotted line is the density of filled traps n t . As the excitation intensity grows the traps are filled, until the density of electrons and holes is large enough that the bimolecular recombination becomes faster than the trapping rate, therefore stopping the accumulation of electrons in the traps. c shows a sketch of the relaxation of optical excitations under steady-state conditions (VB and CB mark the valence and conduction bands, respectively). Full size image Numerical modelling of steady-state PL Figure 5b reports the results of a trap model used to describe the PL response observed under cw excitation. We assumed that an intra-gap level traps one of the two carriers. For exemplification purposes, the sketch in Fig. 5c shows an electron trap. Trapped electrons recombine non-radiatively with holes in the valence bands at later times. This process competes with the direct bimolecular recombination of electrons and holes previously discussed. The corresponding rate equations are explicitly reported in Supplementary Methods (ref. 48 ). We solved these equations under steady-state and quasi-steady-state-pulsed excitations. We found results consistent with experimental findings for both excitation regimes. Here we discuss the main results in steady state. At low-excitation rates, trapping is the most efficient recombination channel for electrons. As electron trapping is a monomolecular process, the conduction electron population scales linearly with the cw laser intensity, n e ∝ I . Conversely, non-radiative recombination of valence holes with trapped electrons is a bimolecular process. Hence, the hole population scales as the square root of the laser intensity, . The steady-state PL intensity then reads [48] : . The bimolecular radiative recombination of free electrons and holes becomes dominant at higher excitation intensities; the power law slowly changes from superlinear to linear owing to the fact that in this excitation regime. At the highest intensities, Auger processes are not anymore negligible and the PL intensity increases sublinearly with laser intensity. The lowest plasma density, n e,h ~2 × 10 18 cm −3 (ref. 17 ), required for optical amplification is achieved for I ~15 kW cm −2 , with an increase by a factor of 3 with respect to the case in which Auger recombination is switched off. The radiative recombination rate of the plasma population is found to be in agreement with the rate of spontaneous emission predicted by the Kubo–Martin–Schwinger law, providing a bimolecular decay constant k b =2.6 × 10 −10 cm 3 s −1 . At moderately high excitation, the population dynamics is governed by the competition of two nonlinear processes, the radiative bimolecular recombination rate and Auger carrier annihilation (Auger constant, γ =2–4 × 10 −28 cm 6 s −1 ). The maximum PL quantum yield is achieved for density range n 0 =0.5–3 × 10 18 cm −3 . We show that Auger processes do not preclude sustaining a plasma population of n ~2 × 10 18 cm −3 under cw excitation; yet, they increase the required laser intensity from I~ 5 kW cm −2 to I~15 kW cm −2 , the latter corresponding to a current density of 5.5 kA cm −2 for electrical injection of the plasma. A legitimate question is what happens to the correlated electron–hole plasma in the high-carrier density regime, where amplified stimulated emission and lasing have been observed. Is light amplification provided by an electron–hole plasma or by a bound-exciton gas? The assumption of thermal equilibrium between bound and ionized excitons implies constant ratio between the square of the free carrier density and the exciton density n X , according to the Saha equation: , where μ X is the effective reduced mass of the exciton with a value μ x =0.15 μ 0 , μ 0 being the electron mass (refs 26 , 29 , 30 ), while T is the temperature of the optical excitations [49] , [50] . Indeed such equilibrium implies that most of the electron–hole pairs are ionized up to n 0 < n eq =2.8 × 10 17 cm −3 . Thermodynamic equilibrium foresees, however, a transition from a conducting plasma [50] , at low electron–hole density, to an insulating excitonic phase for n 0 >2 n eq (details can be found in Supplementary Note 1 ). Such prediction, in combination with the observation that the lasing wavelength is close to the excitonic PL one, has led to interpreting the lasing from perovskite materials as arising from a gas of bound excitons and to speculation about the properties of such excitonic laser [17] , [21] . Contrary to the thermal equilibrium prediction, our analysis of transient PL data in Figs 2 , 3 , 4 indicates, however, that an electron–hole plasma is created at the excitations at which optical gain has been recently reported, namely n las ~2 × 10 18 cm −3 . We infer that the transition to the excitonic gas predicted by the Saha equation is inhibited by nonlinear effects [44] (see Supplementary Fig. 6 ), such as screening and renormalization of the exciton binding energy [51] or simply because the quantum kinetics of the bound and unbound pairs does not allow for reaching the thermal equilibrium between the two gas phases [52] , [53] . Finally, according to a full many-body treatment of the photophysics of a correlated electron–hole plasma, a population of unbound electrons and holes can contribute to the luminescence at ℏ ω = E X , even though no exciton population is really formed [54] . Indeed, this excitonic plasma emission is expected to dominate over the emission of a true exciton population at high temperatures [55] . In the emission process, energy conservation imposes that the extra energy of the recombining electron–hole pair is redistributed among the remaining carriers. A quantum-mechanical analysis thus provides a possible explanation for the intriguing experimental observations of a PL peaked at E X but scaling quadratically with the excitation power. We now address the issue about the minimum density threshold required for achieving light amplification. We still resort to the reference model of non-interacting electron–hole gas as starting point for discussion. In a semiconductor, the crossover between optical absorption and gain occurs at the energy of the electron–hole chemical potential ( μ ) (ref. 42 ). In Fig. 6 , we report μ calculated for a plasma of ionized electron–hole pairs at room temperature. Also reported are the bandgap ( E g ) and exciton ( E X ) transition energies. μ crosses E g at n inv =3 × 10 18 cm −3 ~ n sat (also corresponding to the condition: f e(h) =0.5). n inv represents the threshold for achieving population inversion and thus stimulated emission at the bandgap in a bare electron–hole gas. Exchange and correlation corrections in the evaluation of μ and E g are foreseen to be of the same magnitude and sign [44] . μ − E g should therefore be affected only marginally by many-body effects, and so should n inv . Details on the chemical potential calculation can be found in Supplementary Note 2 . Optical gain can occur also at plasma densities lower than n inv thanks to the scattering events in which an electron–hole pair in the conduction-valence band annihilates, emitting a photon with energy below the chemical potential, ħω < μ ( n )< E X . In these processes, energy is conserved either by a simultaneous phonon emission or by heating of the plasma. 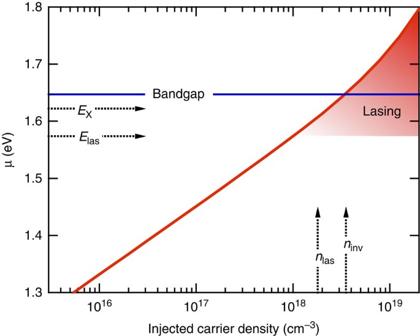Figure 6: Lasing from a free carrier plasma. Optical gain occurs for photon energies below the chemical potential,ħω<μ(n). The chemical potential is calculated for a non-interacting electron–hole plasma (solid-red line). The densityninv=3 × 1018cm−3at whichμcrosses the energy bandgapEgrepresents the ‘reference’ density threshold for light amplification. Lasing can be also achieved belowninv, approximately within a factor of 2 in density, depending on the effective intra-gap density of states and extrinsic optical losses. Amplified spontaneous emission has been recently reported for a density about half of our observed saturation density,. The photon energy at which stimulated emission was observed (Elas=1.574 eV, lower black-dashed arrow) is ~50 meV belowμ(nlas)≈EX(upper black-dashed arrow,EX=1.622 eV), therefore, it satisfies the conditionħω<μbut at the same time meeting the requirement of a non-negligible density of intra-gap states (as inferred from the absorption spectrum reported inFig. 1atElas). Our observations that an electron–hole plasma exists for carrier densities >1018cm−3is consistent with lasing threshold reported in literature, provided lasing action is attributed to the electron–hole plasma instead of a bound-exciton gas (see alsoSupplementary Information). Figure 6 shows that the photon energy at which amplified spontaneous emission has been recently reported satisfies the previous conditions. As the gain cross-section decreases rapidly below the gap, this analysis suggests that n inv represents the ‘reference’ density threshold for light amplification in perovskites films. ‘Reference’ means that lasing can be also achieved below n inv , approximately within a factor of 2 depending on the effective intra-gap density of states and extrinsic optical losses. In Supplementary Fig. 7 , we show that stimulated emission is not allowed for n ~ n inv if the ratio between the populations of bound and unbound excitons follows the Saha equation. Figure 6: Lasing from a free carrier plasma. Optical gain occurs for photon energies below the chemical potential, ħω < μ ( n ). The chemical potential is calculated for a non-interacting electron–hole plasma (solid-red line). The density n inv =3 × 10 18 cm −3 at which μ crosses the energy bandgap E g represents the ‘reference’ density threshold for light amplification. Lasing can be also achieved below n inv , approximately within a factor of 2 in density, depending on the effective intra-gap density of states and extrinsic optical losses. Amplified spontaneous emission has been recently reported for a density about half of our observed saturation density, . The photon energy at which stimulated emission was observed ( E las =1.574 eV, lower black-dashed arrow) is ~50 meV below μ ( n las )≈ E X (upper black-dashed arrow, E X =1.622 eV), therefore, it satisfies the condition ħω < μ but at the same time meeting the requirement of a non-negligible density of intra-gap states (as inferred from the absorption spectrum reported in Fig. 1 at E las ). Our observations that an electron–hole plasma exists for carrier densities >10 18 cm −3 is consistent with lasing threshold reported in literature, provided lasing action is attributed to the electron–hole plasma instead of a bound-exciton gas (see also Supplementary Information ). Full size image In conclusion, we have investigated the excited-state properties of lead halide perovskites under different excitation conditions. We find that optical pumping mainly leads to a population of free carriers, while the population of bound excitons is negligible. We conclude that solar light does not generate an insulating excitonic gas, which necessarily requires a proper heterojunction to split the neutral exciton state and lead to a charge current flow. Coulomb correlations between electrons and holes are, however, important. The binding energy of excitons is found to be 25±3 meV from an analysis of the band-edge absorption conducted in the framework of Elliot’s theory of Wannier excitons. Electron–hole correlations induced by Coulomb interactions do not only yield discrete line absorption at the exciton resonance, but also enhance the oscillator strength of the band-to-band transitions covering the near-infrared to visible electromagnetic spectrum, with a beneficial effect for solar light harvesting. Intra-gap defect states, ubiquitous in solution-processed semiconductors, are also present in organometal halide perovskites and they appear under steady-state excitations, when the rate of radiative bimolecular recombination is negligible. The trap density is not necessarily low and determines the PL lifetime at low light intensities, comparable to those ones provided by sun illumination. Nevertheless, as long as the film is processed in such a way that the mean PL lifetime exceeds several nanoseconds at low excitation, carrier mobility is sufficiently high to guarantee efficient charge collection in the photovoltaic device [19] . Concerning lasing, we conclude that the presence of the electron–hole plasma justifies a low-density threshold, between 1 and 3 × 10 18 cm −3 , for stimulated emission. In this range of excitation, radiative bimolecular decay dominates over carrier trapping by defect states and non-radiative Auger decay, the latter prevailing at higher electron–hole densities. All these features make organometal perovskites very promising for the realization of a solution-processed electrically driven laser. Perovskite synthesis Perovskite solution was prepared by dissolving methylamine iodide (MAI) and PbI 2 or PbCl 2 in dimethylformamide. MAI was prepared by reacting methylamine, 33 wt% in ethanol, with hydroiodic acid (HI), 57 wt% in water. In a typical synthesis, 12 ml of methylamine were added to 50 ml of absolute ethanol and stirred under nitrogen atmosphere at room temperature. Five millilitres of HI were then added by a syringe and left reacting for 2 h (ref. 4 ). The CH 3 NH 3 I salt was crystallized at 50 °C using a rotary evaporator until the powder reached a white-brown colour. The salt was then washed and filtered three times with diethyl ether and dried in vacuum overnight to finally obtain a white powder. All the reactants were purchased from Sigma-Aldrich. Perovskite solutions of MAPbI 3 and MaPbI 3− x Cl x were obtained by dissolving MAI and PbI 2 or PbCl 2 in a 1:1 or 3:1 molar ratio, respectively, in anhydrous dimethyl sulphide in air at room temperature. The solutions were stirred for 12 h before film deposition. Film deposition Films were obtained by spinning the solution, 0.33 M with respect to Pb, on top of soda lime glass substrates at 1,000 r.p.m. for 120 s at room temperature inside a nitrogen-filled glove box. Before deposition the substrates were cleaned with water and soap, rinsed with acetone and ethanol and dried with dry air. The as-deposited films were thermally treated at 100 °C for 1 h on a hot plate inside the glove box to obtain the perovskite structure crystallization. The light yellow fresh films turned brown after a few minutes of treatment thus confirming the crystal formation, but it was necessary to increase the treatment time up to 1 h to achieve the structure stability. Structure and morphology Structural characterization was carried out by analyzing the X-ray diffraction patterns recorded by a Bruker D8-Discover diffractometer for thin films with parallel beam geometry and Cu Kα wavelength. Symmetric ω-2θ scans were obtained using a step size of 0.02° and time per step of 4 s. Film thickness and surface morphology were obtained by atomic force microscopy (AFM) with a NT-MDT Solver P47H-Pro in semicontact mode by a high-resolution non-contact silicon tip. Linear optical properties Optical absorption was measured with films kept in vacuum inside a cold finger cryostat and illuminated by an incandescent tungsten lamp through parabolic mirror optics. An optical chopper was used to modulate the light intensity in time. The transmitted light was dispersed with a grating spectrometer (Acton 2300 series with a 50 g mm −1 , 600 nm blaze grating) and detected by a diode and a lock-in amplifier tuned to the optical chopper frequency. The temperature was varied using liquid nitrogen as a coolant. To measure the PL spectrum, samples were excited with a Nd:Yag cw laser (Spectra Physics Millennia series), 532 nm in wavelength, and the optical emission collected with a grating spectrometer (Acton 2500 series, 600 g mm −1 grating, 500 nm blaze) coupled to a liquid nitrogen cooled CCD camera (Princeton Instruments). Time-resolved PL Two separate laser sources were employed to widen the excitation range available. The low-excitation source was a Ti:sapphire oscillator (Spectra Physics Tsunami) delivering 100-fs-long pulses to a home-made pulse picker to reduce the pulse repetition rate from 80 MHz to 800 Hz (ref. 56 ). The available energy on the sample surface was in the range 0.1–100 pJ per pulse. Higher pulse energies were instead achieved with a regenerative amplifier laser source (Quantronix Integra series), delivering 130-fs-long pulses in KHz repetition rate trains, 1 mJ energy per pulse [57] . Samples were kept in vacuum and the optical emission was dispersed by a spectrometer (Acton 2300 series with a 50 g mm −1 , 600 nm blaze grating) coupled to a streak camera (Hamamatsu C5640). The optical resolution depended on the time range employed on the streak camera and therefore varied from few tens of picoseconds to over 300 ps. cw and quasi-cw PL Samples under vacuum were excited with a 527 nm Nd:Ylf laser either in pulsed mode (1.1 KHz repetition rate, 300 ns duration, achieved with Q-switching) or in cw. The transmitted light was dispersed with a grating spectrometer (Acton 2300 series with a 50 g mm −1 , 600 nm blaze grating) and detected by a diode. How to cite this article: Saba, M. et al. Correlated electron–hole plasma in organometal perovskites. Nat. Commun. 5:5049 doi: 10.1038/ncomms6049 (2014).